Role of dimensional crossover on spin-orbit torque efficiency in magnetic insulator thin films 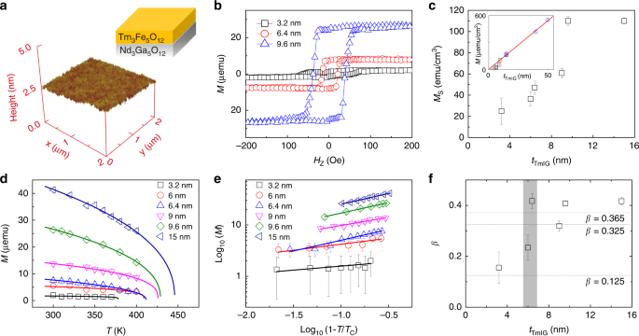Fig. 1 Dimensional crossover of magnetism in TmIG thin films.aAtomic force microscopy image of a 10 nm-thick TmIG film.bMagnetic moment as a function of out-of-plane magnetic field for TmIG thin films with different thicknesses at room temperature.cSaturation magnetization as a function of TmIG thickness at room temperature. The inset shows the areal magnetic moment as a function of TmIG thickness, which indicates a negligible magnetic dead layer.dTotal magnetic moment as a function of temperature for different TmIG thicknesses. The solid lines are power-law fits toM=M0(1 −T/TC)β.elog10(M) vs log10(1 −T/TC) plots from (d) showing the thickness dependence of theβvalues.fCritical exponentβvs TmIG thickness showing a dimensional crossover from 2D to 3D. The dashed lines are theoretical values for 2D Ising (β= 0.125), 3D Ising (β= 0.325), and 3D Heisenberg (β= 0.365) models. The error bars in (c–e) stand for the measurement uncertainty, and the error bar in (f) stands for the fitting uncertainty Magnetic insulators (MIs) attract tremendous interest for spintronic applications due to low Gilbert damping and the absence of Ohmic loss. Spin-orbit torques (SOTs) on MIs are more intriguing than magnetic metals since SOTs cannot be transferred to MIs through direct injection of electron spins. Understanding of SOTs on MIs remains elusive, especially how SOTs scale with the MI film thickness. Here, we observe the critical role of dimensionality on the SOT efficiency by studying the MI layer thickness-dependent SOT efficiency in tungsten/thulium iron garnet (W/TmIG) bilayers. We show that the TmIG thin film evolves from two-dimensional to three-dimensional magnetic phase transitions as the thickness increases. We report the significant enhancement of the measured SOT efficiency as the TmIG thickness increases, which is attributed to the increase of the magnetic moment density. We demonstrate the current-induced SOT switching in the W/TmIG bilayers with a TmIG thickness up to 15 nm. The interplay between heavy metals (HMs) and magnetic insulators (MIs) in heavy metal/magnetic insulator (HM/MI) bilayer systems has attracted tremendous attention from both fundamental research and practical applications [1] , [2] , [3] , [4] . First, the HM/MI bilayer benefits from the low Gilbert damping in the MI. In contrast to magnetic metal, MIs only allow spin information to propagate through magnons, instead of itinerant electrons, due to their large electronic bandgaps. The absence of Ohmic loss from the magnetic layer makes HM/MI bilayers more energy efficient than HM/magnetic metal bilayers. The second advantage of the HM/MI bilayer is that the spin-orbit coupling in the HM or at the HM/MI interface allows the efficient generation of spin-orbit torques (SOTs) on the MI layer through the spin Hall effect (SHE) or Rashba–Edelstein effect [5] , [6] , [7] , [8] , [9] . These SOTs enable efficient manipulation of magnetization dynamics in the MI layer. Although the MI layer is electrically insulating, SOT-driven magnetization dynamics of MIs can be detected through anomalous Hall resistance (AHR) and spin Hall magnetoresistance (SMR) in the HM layer [10] , [11] , [12] , [13] . By probing the AHR, current-induced magnetization switching (CIMS) was observed in both Pt/BaFe 12 O 19 [14] and Pt/Tm 3 Fe 5 O 12 (TmIG) bilayers [15] , [16] . However, whether SOTs in Pt/MI bilayers are from SHE remains ambiguous due to the potential existence of the Rashba–Edelstein effect [16] . It remains unclear whether the switching direction will be opposite when we utilize HMs with opposite spin Hall angles. Moreover, the observed damping-like SOT efficiency ( ξ DL ) in the Pt/TmIG that is responsible for switching is still much lower than those in the Pt/ferromagnetic metals (FMs) [15] , [17] , [18] . To understand the origin of SOTs and to increase the value of ξ DL in HM/MI bilayers, we utilize a HM with a large spin Hall angle opposite to that of Pt in a HM/MI bilayer, demonstrate magnetization switching, and analyze the contributions to the SOT. 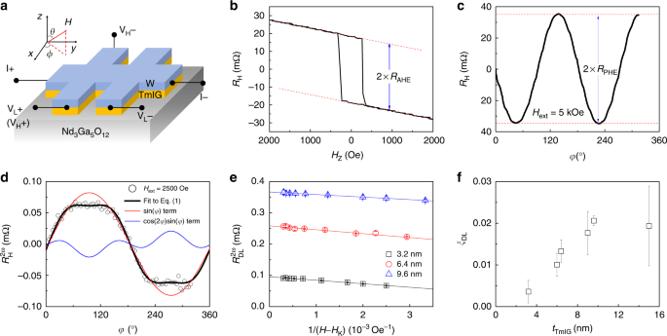Fig. 2 Spin transport and SOT measurements in the W/TmIG bilayers.aExperimental setup for measuring resistance, SOT, and current-induced magnetization switching.bHall resistance as a function of an out-of-plane magnetic field for the W (5 nm)/TmIG (9.6 nm), where AHE is observed as the sharp square hysteresis loop.cHall resistance as a function of a rotating in-plane constant magnetic field (5 kOe) for the W (5 nm)/TmIG (9.6 nm), where SMR-induced PHE is observed.dSecond-harmonic Hall resistance as a function of in-plane azimuthal angle for the external magnetic field 2500 Oe for the W (5 nm)/TmIG (3.2 nm), where the black curve is the fit to Eq. (1). Both cos 2φsinφ(blue curve) and sinφ(red curve) angle dependencies are revealed.eExtracted damping-like torque contribution as a function of the inverse of external magnetic field subtracting the anisotropy field. The large intercepts are the spin Seebeck resistance.fDamping-like spin-orbit torque efficiency as a function of TmIG thickness. The error bar stands for the fitting uncertainty In this article, we study the ξ DL and CIMS in tungsten (W)/TmIG heterostructures with different TmIG layer thicknesses ( t TmIG ). The thickness dependence of the damping-like SOT allows us to understand the interplay between spin current and magnetism in TmIG. Here, W is chosen since it is reported to give the largest spin Hall angle among elemental HMs and its sign is opposite to that of Pt [19] . When the TmIG film thickness is reduced from 15 to 3.2 nm, the effective exchange coupling is strongly reduced due to long-wavelength thermal fluctuations, resulting in a dimensional crossover from three-dimension-like to two-dimension-like magnetic phase transitions. We quantify ξ DL by using second-harmonic Hall measurements [20] , [21] . The ξ DL increases with the t TmIG in W/TmIG bilayers; this is attributed to the enhanced magnetic moment density due to suppression of thermal fluctuations. We then demonstrate the CIMS in W/TmIG bilayers up to t TmIG = 15 nm; for t TmIG = 15 nm, the switching current density is as low as 8 × 10 10 A/m 2 . The estimated current switching efficiency enhances as t TmIG increases, which is consistent with the increase of ξ DL with t TmIG . Importantly, the switching direction of our W/TmIG devices is indeed opposite to that of the Pt/TmIG device [15] ; this contrast confirms the important role of SHE in CIMS of MIs. Dimensional crossover of magnetism To access SOT and realize CIMS, we prepare high-quality TmIG thin films with different t TmIG and characterize their magnetic properties. These TmIG(111) thin films were grown on substrate Nd 3 Ga 5 O 12 (111) by pulsed laser deposition [13] . All TmIG thin films show an atomically flat surface with mean roughness as low as 0.1 nm (Fig. 1a ), providing a sharp interface for efficient spin momentum transfer. The Gilbert damping of TmIG thin films increases as the thickness decreases (see Supplementary Note 1 ). The large lattice mismatch between the TmIG and the Nd 3 Ga 5 O 12 provides the tensile strain to generate perpendicular magnetic anisotropy in all TmIG thin films. The nature of perpendicular magnetic anisotropy is confirmed using magnetization hysteresis loops of TmIG thin films as a function of an out-of-plane magnetic field (Fig. 1b ), from which we can determine saturation magnetization ( M S ). We observe a strong t TmIG dependence of the M S at room temperature (Fig. 1c ); the M S reduces significantly from the bulk M S (110 emu/cm 3 ) [22] with decreasing film thickness. Note that the estimated dead layer thickness is less than 1 nm (see Fig. 1c inset and Supplementary Note 2 ), which also suggests a sharp interface between TmIG and substrate [23] . The reduction of the M S at room temperature is attributed to finite size effect, strong thermal fluctuation and strong surface modification effect in ultrathin magnetic films [24] , [25] , [26] . Following ref. [25] , we extract the critical exponents β for magnetic phase transitions in these TmIG thin films using temperature dependence of magnetic moment ( M – T ). The M – T curves follow the M = M 0 (1 − T / T C ) β (Fig. 1d ), where zero-temperature magnetic moment ( M 0 ) and Curie temperature ( T C ) are fitting parameters. The t TmIG -dependent β is better illustrated using log–log plots as shown in Fig. 1e and the results are summarized in Fig. 1f . We see a clear increase of β from 0.16 ± 0.06 to 0.42 ± 0.02 when the t TmIG increases from 3.2 to 15 nm, where the uncertainty is coming from the fitting. This increase of β suggests a dimensional crossover from two-dimension-like to three-dimension-like magnetism since 2D Ising model and 3D Heisenberg model predict β to be 0.125 and 0.365, respectively [26] , [27] . The dimensional crossover happens at around 6 nm, which is one order of magnitude larger than the typical transition thickness around 1 nm for magnetic metals [25] , [26] , [27] . In the following sections, we point out that the reduction of M S due to dimensional crossover has a major influence on the magnitude of the SOT and switching efficiency, which has been neglected in the previous experiments. Fig. 1 Dimensional crossover of magnetism in TmIG thin films. a Atomic force microscopy image of a 10 nm-thick TmIG film. b Magnetic moment as a function of out-of-plane magnetic field for TmIG thin films with different thicknesses at room temperature. c Saturation magnetization as a function of TmIG thickness at room temperature. The inset shows the areal magnetic moment as a function of TmIG thickness, which indicates a negligible magnetic dead layer. d Total magnetic moment as a function of temperature for different TmIG thicknesses. The solid lines are power-law fits to M = M 0 (1 − T / T C ) β . e log 10 ( M ) vs log 10 (1 − T / T C ) plots from ( d ) showing the thickness dependence of the β values. f Critical exponent β vs TmIG thickness showing a dimensional crossover from 2D to 3D. The dashed lines are theoretical values for 2D Ising ( β = 0.125), 3D Ising ( β = 0.325), and 3D Heisenberg ( β = 0.365) models. The error bars in ( c – e ) stand for the measurement uncertainty, and the error bar in ( f ) stands for the fitting uncertainty Full size image SOT measurement To perform resistance, SOT, and CIMS measurements, we fabricate W(5 nm)/TmIG( t TmIG ) thin films into Hall bar devices (Fig. 2a ). By using four-probe resistance measurements in different Hall bar devices, we determine the W resistivity to be 155 ± 15 µΩ·cm, where the uncertainty is estimated from the multiple (>20) device measurements. According to ref. [19] , pure α-W has resistivity around 20 µΩ·cm, and 6 nm-thick W with mixed α- and β-phases has a resistivity as high as 170 µΩ·cm. So, most likely, our 5 nm-thick W thin films have mixed α- and β-phases. The AHR in the W/TmIG is accurately determined by the sharp anomalous Hall hysteresis at low fields (Fig. 2b ). The transverse planar Hall resistance (PHR) accompanying the longitudinal SMR is measured by rotating the magnetization in the xy -plane (Fig. 2c ). The observation of sizeable AHR and PHR (SMR) indicates that there is a significant spin current being transmitted across the W/TmIG interface or a sizable spin mixing conductance [11] (see Supplementary Note 3 ). Fig. 2 Spin transport and SOT measurements in the W/TmIG bilayers. a Experimental setup for measuring resistance, SOT, and current-induced magnetization switching. b Hall resistance as a function of an out-of-plane magnetic field for the W (5 nm)/TmIG (9.6 nm), where AHE is observed as the sharp square hysteresis loop. c Hall resistance as a function of a rotating in-plane constant magnetic field (5 kOe) for the W (5 nm)/TmIG (9.6 nm), where SMR-induced PHE is observed. d Second-harmonic Hall resistance as a function of in-plane azimuthal angle for the external magnetic field 2500 Oe for the W (5 nm)/TmIG (3.2 nm), where the black curve is the fit to Eq. ( 1 ). Both cos 2 φ sin φ (blue curve) and sin φ (red curve) angle dependencies are revealed. e Extracted damping-like torque contribution as a function of the inverse of external magnetic field subtracting the anisotropy field. The large intercepts are the spin Seebeck resistance. f Damping-like spin-orbit torque efficiency as a function of TmIG thickness. The error bar stands for the fitting uncertainty Full size image We quantify ξ DL by using the second-harmonic analysis of both AHR and PHR ( R AHE and R PHE ) [20] , [21] . The second-harmonic Hall resistance ( \(R_{\mathrm{H}}^{2\omega }\) ) in a single domain subjected to an in-plane magnetic field can be written as [21] , [28] 
    R_H^2ω = 1.5pt R_FL^2ωcos 2φsinφ + R_DL^2ωsinφ = R_PHEH_FL/| H_ext|cos 2φsinφ
     + ( R_AHE/2H_DL/| H_ext| - H_K + R_SSE)sinφ
 (1) where H K and H ext are perpendicular magnetic anisotropy effective field and in-plane external field, respectively. In Eq. ( 1 ), \(R_{{\mathrm{FL}}}^{2\omega }\) and \(R_{{\mathrm{DL}}}^{2\omega }\) are the peak values of cos 2 φ sin φ and sin φ components in \(R_{\mathrm{H}}^{2\omega }\) , which are field-like SOT and damping-like SOT contributions, respectively. H FL and H DL are the current-induced field-like and damping-like effective fields, respectively. For example, when the H ext = 2500 Oe, we observe significant contributions from both damping-like and field-like SOTs, as reflected by the cos 2 φ sin φ and sin φ angle dependencies (see Fig. 2d and Supplementary Note 4 ). According to Eq. ( 1 ), slopes of linear fits to the \(R_{{\mathrm{DL}}}^{2\omega }\) as a function of 1/( H ext − H K ) (Fig. 2e ) give the information about H DL , and the intercepts are the spin Seebeck resistances (or voltages), which is field-independent in the single domain case (see Eq. ( 1 )) [21] , [29] . We calculate ξ DL using \(\xi _{{\mathrm{DL}}} = \frac{{2eM_{\mathrm{S}}t_{{\mathrm{TmIG}}}H_{{\mathrm{DL}}}}}{{\hbar J_{{\mathrm{ac}}}}}\) [6] , where e is the electron charge, ħ is the reduced Planck constant, and J ac is the applied current density. We observe a characteristic increase of ξ DL as t TmIG increases with a saturation length of 10 nm (see Fig. 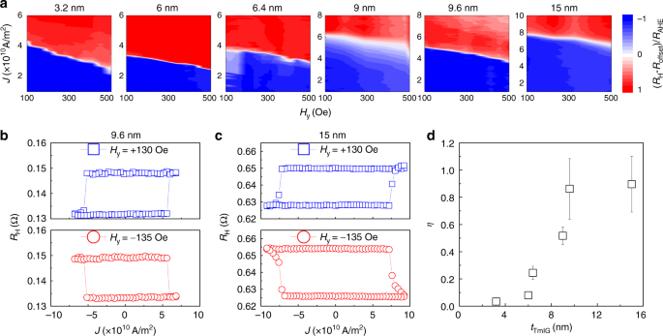Fig. 3 Current-induced magnetization switching in W/TmIG with different TmIG thicknesses.aSwitching phase diagram for TmIG with thicknesses from 3.2 to 15 nm, where the external field is along the current direction.Roffsetis device-dependent Hall resistance offset. For instances,b,cshow the current-induced switching for TmIG with thickness 9.6 and 15 nm, respectively, in the presence of a magnetic field along and against the current direction. The switching is done by applying a 5 ms pulse with varying current amplitude.dTmIG thickness-dependent current switching efficiency, which is estimated from the depinning (coercive) field over switching current density in the zero-external field limit. The error bar originates from the multiple (>3) device measurements 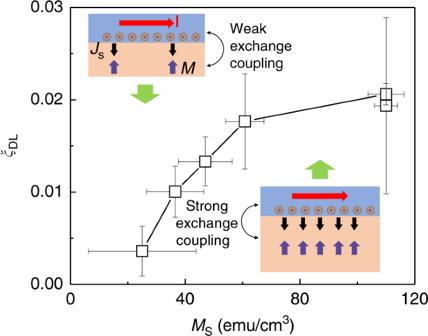Fig. 4 Role of TmIGMSon theξDL.ξDLis proportional to theMSsquared as shown in the text when theMSis small due to strong thermal fluctuation and surface modification effect. Insets show two cases: in the left inset, the magnetic moment density is small and thus the interfacial exchange interaction is weak, resulting in a small spin current injection; in the right inset, the magnetic moment density is large due to suppressed thermal fluctuation and thus the interfacial exchange interaction is strong, resulting in a large spin current injection. Definitions of the error bars forMSandξDLare given in Figs.1,2, respectively 2f ). Similarly, previous experiments have revealed a saturation length around 1 nm in FM heterostructures [18] , [30] , [31] . This saturation length is very close to the measured penetration depth of transverse spin current for FMs using spin pumping technique [32] , [33] , [34] . Thus, the saturation length has been interpreted as an indicator of penetration depth [33] , [34] . However, for our MI TmIG thin films, the scenario becomes complex since the electron spin cannot directly tunnel into the MI and the magnetism of MI thin films is strongly dependent on the MI thickness (Fig. 1 ). Note that the SOT efficiency ( ξ DL ~0.02) in our W/TmIG (≥9 nm) devices is smaller than that in β-W/CoFeB (ξ DL ~0.3) [19] . There are two possible reasons. First, our W thin films are in mixed phases, which have a smaller spin Hall angle. Second, the material interfaces in W/magnetic metal and W/MI bilayers could be very different [17] , which requires further investigations. SOT switching After quantifying the SOT efficiency, we perform the CIMS experiments for W/TmIGs with different t TmIG . The switching is achieved in all devices with t TmIG up to 15 nm and the switching phase diagrams are summarized in Fig. 3a . In the presence of an external field along the + y direction, a sufficiently large charge current along the + y direction will cause magnetization (AHR) switching from the + z direction to the − z direction (negative to positive). The required amount of charge current to flip the magnetization decreases as the external field increases. When we apply a sufficiently large charge current along the − y direction while keeping the external field along the + y direction, the magnetization (AHR) is switched from the − z direction to the + z direction (positive to negative) (upper panels in Fig. 3b, c ). For the same current direction, the switching direction is opposite when we reverse the external field direction (lower panels in Fig. 3b, c ). All of the above facts agree with the picture of SOT-driven magnetization switching. Note that the switching current density is as low as 6 × 10 10 A/m 2 for the W (5 nm)/TmIG (9.6 nm) (Fig. 3b ), which is three times smaller than the Pt (5 nm)/TmIG (8 nm) case [15] . This suggests that W enables more energy efficient magnetization switching. Fig. 3 Current-induced magnetization switching in W/TmIG with different TmIG thicknesses. a Switching phase diagram for TmIG with thicknesses from 3.2 to 15 nm, where the external field is along the current direction. R offset is device-dependent Hall resistance offset. For instances, b , c show the current-induced switching for TmIG with thickness 9.6 and 15 nm, respectively, in the presence of a magnetic field along and against the current direction. The switching is done by applying a 5 ms pulse with varying current amplitude. d TmIG thickness-dependent current switching efficiency, which is estimated from the depinning (coercive) field over switching current density in the zero-external field limit. The error bar originates from the multiple (>3) device measurements Full size image The switching direction driven by current-induced SOTs is consistent with the sign of the spin Hall angle of W, and it is opposite to that in the Pt/TmIG bilayer [15] . Therefore, our work strongly suggests the dominant role of the SHE in the generation of SOTs and CIMS in HM/MI bilayers. However, we do notice that there could be an interfacial Rashba–Edelstein effect at the W/TmIG interface contributing to the SOTs by comparative analyses of SOTs and SMR (AHR) (see Supplementary Note 5 ). To quantitatively compare the switching efficiency of W/TmIG devices with different t TmIG , we define an effective switching efficiency as \(\eta = \frac{{2eM_{\mathrm{S}}t_{{\mathrm{TmIG}}}H_{\mathrm{P}}}}{{\hbar J_{{\mathrm{sw}}}(H_{\mathrm{y}} \to 0)}}\) [35] , where H P is the domain wall depinning field estimated from the coercive field (see Supplementary Note 6 ) and J sw ( H y → 0) is the zero-field limit of current density in the switching phase diagram. This formula is chosen because the CIMS is achieved through domain nucleation and domain wall motion in the Hall bar devices due to the large scale of our Hall bar devices, of which the channel width is 20 µm [36] . We observe a dramatic increase of η with t TmIG (Fig. 3d ), for which we consider two reasons. First, the ξ DL increases with t TmIG , which means that the same amount of charge current in the W layer generates stronger damping-like SOT on the TmIG layer. Thus, the increase of ξ DL contributes to a lower J sw and thus a larger η . Second, the Joule heating effect becomes much more significant when a larger charge current is applied, which is the case for switching a thicker TmIG. Joule heating causes reduction of thermal stability through decreasing the M S and H P ; these two values will be smaller than those measured at the low current limit. Therefore, the M S and H P used to calculate η are overestimated, leading to a larger η . Here, we discuss the mechanism for the MI thickness dependence of ξ DL . We propose that ξ DL depends on M S when M S of the thin films is well below the corresponding bulk value. The Landau–Lifshitz–Gilbert equation in the presence of damping-like SOT can be written as 
    M_S t_Mdm̂/dt = - γ M_St_Mm̂×H⃗_eff + α M_St_Mm̂×dm̂/dt
     + γ J_Cξ _DLħ/2e( m̂×σ̂×m̂)
 (2) where \(\hat m\) is the unit vector of magnetization, \(\hat \sigma\) is the unit vector of current-induced spin polarization, γ is the gyromagnetic ratio, α is the Gilbert damping, t M is the thickness of the magnetic layer, J C is the charge current density, and \(\vec H_{{\mathrm{eff}}}( = \vec H_{\mathrm{K}} + \vec H_{{\mathrm{ext}}})\) is the total effective magnetic field acting on the magnetization. The last term on the right-hand side of Eq. ( 2 ) arises due to the absorption of transverse spin current by the magnet, which is referred to as the current-induced damping-like (dissipative) SOT. Its strength is parameterized by dimensionless efficiency parameters ξ DL . The origin of the SOT can be understood in a simple microscopic picture as follows. A charge current at the HM and ferromagnet interface induces an accumulation of spin density, \(\rho \hat \sigma\) , due to the finite spin-orbit interaction (for example, by SHE or Rashba–Edelstein effect). Here, ρ is the magnitude of the spin density, which is proportional to the strength of the spin-orbit interaction. This spin density interacts with the ferromagnet via exchange interaction, of the form \(U_{{\mathrm{ex}}} \sim \rho M_{\mathrm{S}}\hat m \cdot \hat \sigma\) , enabling the absorption of the spin current by the ferromagnet. In the perturbative treatment, the spin current absorbed by the ferromagnet can be obtained up to second order in the exchange interaction to yield the damping-like SOT with \(\xi _{{\mathrm{DL}}}\sim M_{\mathrm{S}}^2\) [37] . The positive correlation between ξ DL and M S is referred as the M S -effect; it has also been theoretically studied in the frame of spin pumping effect (in Appendix B of ref. [38] ), which is the Onsager reciprocal process of the spin torque effect. The increase of spin mixing conductance with M S is consistent with the calculation from first principles [39] when the surface modification effect presents in the ultrathin regime [26] . Our experiments are the demonstrations of the M S -effect; we show that as the thickness increases, the SOT efficiency significantly increases with M S in the low M S -regime (see Fig. 4 ), which is in qualitative agreement with the M S -effect. Also, we show that as the temperature decreases, the SOT efficiency increases with M S , due to suppression of thermal fluctuations (see Supplementary Note 7 ). Intuitively, as the magnetic moment density ( M S ) increases, the interfacial exchange interaction is enhanced, which allows more spin current to pass through the interface. As the thickness increases, the SOT efficiency saturates earlier than M S , around half of the bulk magnetization (60 emu/cm 3 ), which suggests that the SOT is determined by the local magnetization that is saturated at a smaller thickness than the global magnetization M S . Our experiments show the need for further investigation of the interaction between ultrathin magnetic films and HMs, which would include the spin physics of dimensional crossover. Fig. 4 Role of TmIG M S on the ξ DL . ξ DL is proportional to the M S squared as shown in the text when the M S is small due to strong thermal fluctuation and surface modification effect. Insets show two cases: in the left inset, the magnetic moment density is small and thus the interfacial exchange interaction is weak, resulting in a small spin current injection; in the right inset, the magnetic moment density is large due to suppressed thermal fluctuation and thus the interfacial exchange interaction is strong, resulting in a large spin current injection. Definitions of the error bars for M S and ξ DL are given in Figs. 1 , 2 , respectively Full size image In summary, we have systematically studied the dimensional crossover of magnetism and its effect on SOTs in ultrathin MI films with perpendicular magnetic anisotropy. The characteristic increase of SOT efficiency with the MI thickness can be understood from the enhancement of magnetic moment density and the suppression of thermal fluctuations. In addition, we have realized CIMS in W/TmIG devices with t TmIG up to 15 nm. The switching current density for W/TmIG devices is lower or comparable with these for HM/FM despite the fact that the saturated ξ DL is estimated to be only around 0.02 at this stage, which is much less than the 0.3 that is estimated for W in W/CoFeB bilayers [19] . Further improvement of the ξ DL could be done by spin mixing conductance matching [40] and surface treatment [41] . Our results presented here show the great potential of ultrathin MI-based spintronics. Materials growth and characterization All TmIG(111) films were grown on Nd 3 Ga 5 O 12 (111) by pulsed laser deposition [13] before transferring to a magnetron sputtering chamber in the ambient condition. At room temperature, we deposited a 5 nm-thick W layer on top of TmIG followed by subsequent deposition of MgO (2 nm)/TaO x (3 nm) layers to protect W from oxidization. Magnetization hysteresis loops as a function of an out-of-plane magnetic field were measured by a vibrating sample magnetometer and a superconducting quantum interference device. The nominal thin film area is 5 × 5 mm 2 . Devices fabrication and characterization The films were patterned into Hall bar devices (Fig. 2a ) by using standard photolithography and dry etching for the resistance, SOT, and switching measurements. The channel width is 20 µm, and the distance between two neighboring Hall contacts is 26 µm. We measured the second-harmonic Hall resistance by applying I ac,r.m.s = 1 mA ( J ac,r.m.s = 10 10 A/m 2 ) with a frequency ω /2 π = 195.85 Hz. The magnetic field and angle controls were done in a physical properties measurement system. The CIMS experiments were performed in the ambient environment by applying a pulse current with 5 ms pulse width and reading Hall voltage subsequently.